Resonant magnetic exciton mode in the heavy-fermion antiferromagnet CeB6 Resonant magnetic excitations are recognised as hallmarks of unconventional superconductivity in copper oxides, iron pnictides and heavy-fermion compounds. Model calculations have related these modes to the microscopic properties of the pair wave function, but the mechanisms of their formation are still debated. Here we report the discovery of a similar resonant mode in the non-superconducting antiferromagnetic heavy-fermion metal CeB 6 . Unlike conventional magnons, the mode is non-dispersive and is sharply peaked around a wave vector separate from those characterising the antiferromagnetic order. It is likely associated with a co-existing order parameter of the unusual antiferro-quadrupolar phase of CeB 6 , which has long remained hidden to neutron-scattering probes. The mode energy increases continuously below the onset temperature for antiferromagnetism, in parallel to the opening of a nearly isotropic spin gap throughout the Brillouin zone. These attributes are similar to those of the resonant modes in unconventional superconductors. This unexpected commonality between the two disparate ground states indicates the dominance of itinerant spin dynamics in the ordered low-temperature phases of CeB 6 and throws new light on the interplay between antiferromagnetism, superconductivity and 'hidden' order parameters in correlated-electron materials. In copper-oxide, iron-pnictide and heavy-fermion superconductors, antiferromagnetic (AFM) order can be induced by changes in pressure, doping level or magnetic field. Theories of magnetically mediated Cooper pairing inspired by this observation have received strong support from neutron-scattering experiments that revealed resonant magnetic excitations in the superconducting states of all of these compounds [1] , [2] , [3] , [4] , [5] , [6] . The resonant modes share a common set of characteristics. They are sharp in both energy and momentum, unlike the incoherent particle-hole excitations in a metal, and are located below the superconducting gap, 2Δ. As model calculations indicate that the spectral weight and momentum-space structure of the resonant modes contain essential information about the pairing interaction [1] , [3] , [6] , pairing symmetry [7] , [8] , [9] , [10] and condensation energy [11] of the superconducting state, research on their origin remains at the frontier of the quest for a comprehensive description of unconventional superconductivity. Here we report inelastic neutron-scattering (INS) experiments that reveal a resonant mode with identical characteristics in the non-superconducting heavy-fermion metal CeB 6 , which has been intensely investigated because of its intriguing phase behaviour [12] , [13] , [14] on the background of an exceptionally simple crystal structure and chemical composition. The electronic states near the Fermi level of CeB 6 are composed of localised cerium-4 f 1 levels hybridised with itinerant cerium-5 d and boron-2 p electrons [15] , [16] , closely analogous to those of the superconductors CeCoIn 5 and CeCu 2 Si 2 , where prominent resonant modes have been reported [4] , [6] . In contrast to these superconducting compounds, however, CeB 6 exhibits AFM order below T N =2.3 K [17] . It is preceded by another phase transition at T Q =3.2 K, whose order parameter has long remained hidden to standard experimental probes such as neutron diffraction [12] , [13] . Theoretical work [18] , [19] has attributed both transitions to interactions between the multipolar moments of the Ce-4 f electrons mediated by the itinerant conduction electrons, which break the large ground-state degeneracy of the cerium ions in their cubic crystal field and stabilise an antiferro-quadrupolar (AFQ) order [20] , [21] , [22] . Recent transport, thermodynamic and neutron diffraction experiments [23] , [24] , [25] , [26] , [16] have revealed deviations from predictions of this interacting multipole model of magnetism in CeB 6 . In particular, weak Bragg intensity has been detected by spin-polarised neutron scattering at the AFQ wave vector, although the concept of quadrupolar ordering forbids such an intensity in the absence of external magnetic fields [12] , [13] , so that it is hidden to the elastic neutron scattering. This observation has been ascribed to the magnetic response of the itinerant Ce-5 d electrons [16] . Our discovery of a magnetic resonant mode for T < T N confirms a more pronounced influence of itinerant electrons on the magnetic properties of CeB 6 than anticipated by the prevailing theory, and establishes a surprising correspondence to unconventional superconductivity. Elastic neutron scattering We start the presentation of our data by comparing the AFM and AFQ magnetic Bragg intensities, measured at and , respectively, in Fig. 1 . From the different onset temperatures of the elastic signals, it is clear that they represent distinct order parameters. The elastic intensity at Q AFQ is more than an order of magnitude weaker than the AFM Bragg intensity, and exhibits only a weak suppression below T N , indicating that both order parameters coexist in the AFM phase. 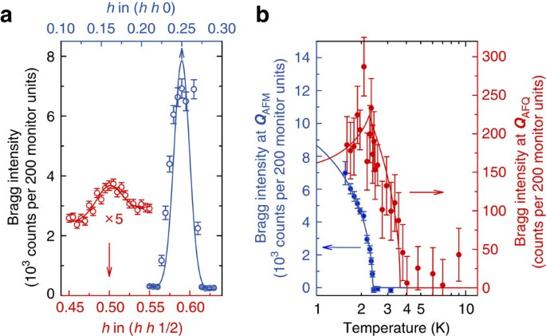Figure 1: Bragg peaks associated with the AFQ and AFM order parameters. (a) Comparison of the elastic signals measured at(left) and(right) atT=1.6 K. The AFQ intensity has been multiplied by a factor of 5 for clarity. (b) Temperature dependence of the corresponding peak intensities that vanish atTQandTN, respectively. The solid lines are guides to the eyes. The error bars in this and all the following figures correspond to one s.d. of the count rate. Figure 1: Bragg peaks associated with the AFQ and AFM order parameters. ( a ) Comparison of the elastic signals measured at (left) and (right) at T =1.6 K. The AFQ intensity has been multiplied by a factor of 5 for clarity. ( b ) Temperature dependence of the corresponding peak intensities that vanish at T Q and T N , respectively. The solid lines are guides to the eyes. The error bars in this and all the following figures correspond to one s.d. of the count rate. Full size image Manifestation of the resonant magnetic exciton mode To give an overview of the inelastic-scattering signal, we present in Fig. 2 unprocessed INS intensity maps of the ( hhl ) plane in reciprocal space, measured in the AFM low-temperature phase ( T =1.6 K) at fixed energy transfers of ħω =0.25, 0.5 and 0.9 meV. An intense peak centered at Q AFQ dominates the spectrum at ħω =0.5 meV ( Fig. 2a ). It can be observed at the two equivalent R points and covered by the measurement, which are additionally connected by weaker streaks of intensity that surround the M point. Intensity maps at both lower ( Fig. 2b ) and higher ( Fig. 2c ) energies reveal greatly reduced intensities. 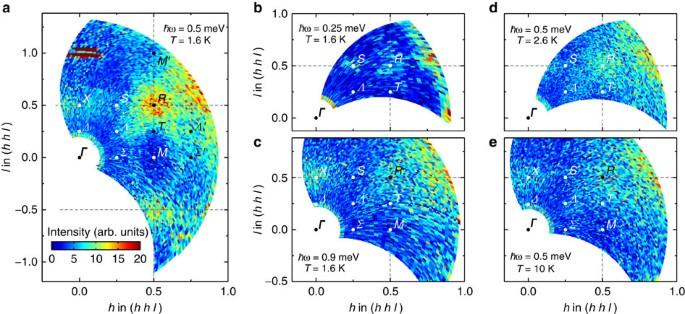Figure 2: Reciprocal space maps. (a) Inelastic signal along the (hhl) plane in reciprocal space, measured in the low-temperature AFM phase (T=1.6 K) at 0.5 meV energy transfer. The labels represent different high-symmetry points, and the dashed lines mark Brillouin zone boundaries. (b,c) The same at lower (0.25 meV) and higher (0.9 meV) energies, respectively. (d,e) The same at two elevated temperatures (2.6 K and 10 K). All panels share the same colour scale. Figure 2: Reciprocal space maps. ( a ) Inelastic signal along the ( hhl ) plane in reciprocal space, measured in the low-temperature AFM phase ( T =1.6 K) at 0.5 meV energy transfer. The labels represent different high-symmetry points, and the dashed lines mark Brillouin zone boundaries. ( b,c ) The same at lower (0.25 meV) and higher (0.9 meV) energies, respectively. ( d,e ) The same at two elevated temperatures (2.6 K and 10 K). All panels share the same colour scale. Full size image The strong concentration of magnetic spectral weight around isolated points in energy-momentum space is markedly different from the continuously dispersive spin waves in conventional antiferromagnets, but closely similar to the behaviour of the resonant modes observed in superconducting compounds below their respective transition temperatures, T c [1] , [2] , [3] , [4] , [5] , [6] . Moreover, the mode is not centred at the S or Σ points characterising the AFM order, where the magnetic intensity is much weaker, but at the R point that reflects the 'hidden' AFQ phase. In Fig. 2b , one can also observe weak intensity near the S point that originates from conventional spin-wave excitations associated with the AFM phase. At 0.25 meV, their intensity is comparable in magnitude to the signal at the R point, whereas at the resonance energy of 0.5 meV ( Fig. 2a ), the latter is enhanced more than two-fold, although the spin-wave intensity at the S point can no longer be observed within the statistical noise. Temperature dependence As the temperature is increased above T N , the strong intensity at the R point is first sharply suppressed already in the AFQ phase ( Fig. 2d ) and then continues to diminish gradually with a further temperature increase far into the paramagnetic phase ( Fig. 2e ). At T =1.6 K, the resonant mode is sharp in energy ( Fig. 3a ) and is characterised by the intrinsic (resolution-corrected) full width at half maximum of ~0.2 meV. It is followed by a weaker second peak centred around 1.1 meV, with the full width at half maximum of ~0.6 meV. For T > T N , the 0.5 meV peak transforms into a quasi-elastic response [27] , [28] that is typical for the paramagnetic state of heavy-fermion metals [5] , [6] . A similar behaviour, but with an exciton mode that is weaker and not as sharp in energy, can also be observed at other points throughout the Brillouin zone ( Fig. 3b,c ). We can therefore associate the formation of the resonant peak with the opening of a spin gap in the low-energy part of the quasielastic spectrum upon cooling and the consequent spectral-weight transfer from below ~0.35 meV to higher energies. In contrast, the second peak at 1.1 meV at the R point is nearly insensitive to T N and possibly arises from a low-energy crystal-field excitation similar to those previously studied in the AFQ phase. 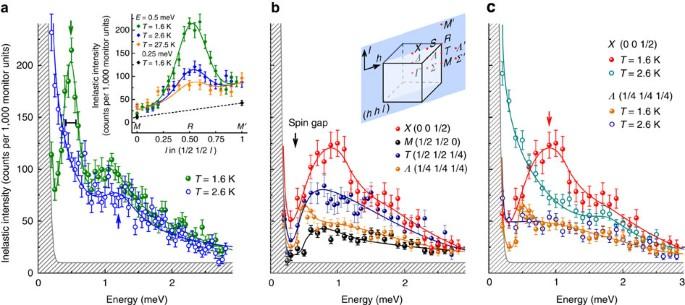Figure 3: Unprocessed INS data. (a) Energy dependence of the INS signal in the AFQ (empty symbols) and AFM (filled symbols) states, measured at thepoint, where the intensity is maximised. Exciton peaks are marked by arrows. The horizontal black bar inside the peak shows the experimental energy resolution, the hatched region represents background intensity, and the lines are guides to the eyes. The inset shows constant energy scans across the peak maximum (ħω=0.5 meV) along theMRM′ line at different temperatures; the dashed line is the background level suggested by the intensity minima atandwithin the spin gap (ħω=0.25 meV). (b) Low-temperature (T=1.6 K) energy scans for theX, M, Tand Λ points. The location of the scattering plane and the naming of high-symmetry points in the cubic Brillouin zone are shown in the inset. (c) Comparison of the energy scans measured at theXand Λ points above and belowTN. [29] , [28] Figure 3: Unprocessed INS data. ( a ) Energy dependence of the INS signal in the AFQ (empty symbols) and AFM (filled symbols) states, measured at the point, where the intensity is maximised. Exciton peaks are marked by arrows. The horizontal black bar inside the peak shows the experimental energy resolution, the hatched region represents background intensity, and the lines are guides to the eyes. The inset shows constant energy scans across the peak maximum ( ħω =0.5 meV) along the MRM ′ line at different temperatures; the dashed line is the background level suggested by the intensity minima at and within the spin gap ( ħω =0.25 meV). ( b ) Low-temperature ( T =1.6 K) energy scans for the X, M, T and Λ points. The location of the scattering plane and the naming of high-symmetry points in the cubic Brillouin zone are shown in the inset. ( c ) Comparison of the energy scans measured at the X and Λ points above and below T N . Full size image The detailed temperature dependence of the resonant mode is illustrated in Fig. 4 , where we plot the imaginary part of the dynamical spin susceptibility, χ ″( Q AFQ , ω ), obtained by correcting the background-subtracted INS signal for the thermal population factor. In Fig. 4a , one sees that the mode gradually broadens and shifts towards lower energies upon warming, following the order-parameter-like trend shown in the inset of Fig. 4b . This behaviour is again strikingly similar to the one of the resonant mode in unconventional superconductors ( Fig. 4c ). For T > T N , the quasielastic signal continues to diminish in intensity with increasing temperature ( Fig. 4b ). Constant-energy scans in the inset of Fig. 3a demonstrate that it always remains peaked at the commensurate wave vector Q AFQ , where the resonant mode develops below T N . 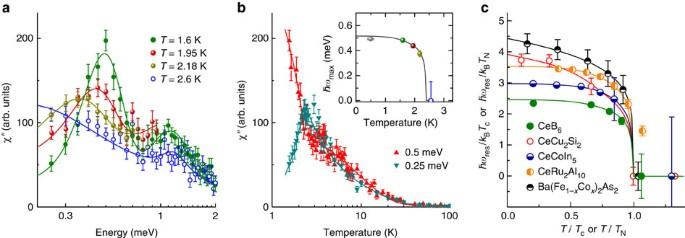Figure 4: Temperature dependence. (a) Imaginary part of the dynamic spin susceptibility,χ″(QAFQ,ω), at various temperatures, illustrating the gradual development of the spin-exciton peak below the AFM transition. The lines are visual guides. (b) Temperature dependence ofχ″(QAFQ,ω) at the peak maximum (ħω=0.5 meV) and within the spin gap (ħω=0.25 meV). The inset shows the exciton energy versus temperature, determined from the position of the peak maximum, ħωmax, in panel (a). (c) Comparison of the normalised resonance energies,ħωres/kBTN(orTc), plotted versus reduced temperature,T/TN(orTc), in CeB6, in several unconventional superconductors3,4,6, and in the low-temperature phase of CeRu2Al10(ref.35). The lines are guides to the eyes. Figure 4: Temperature dependence. ( a ) Imaginary part of the dynamic spin susceptibility, χ ″( Q AFQ , ω ), at various temperatures, illustrating the gradual development of the spin-exciton peak below the AFM transition. The lines are visual guides. ( b ) Temperature dependence of χ ″( Q AFQ , ω ) at the peak maximum (ħ ω =0.5 meV) and within the spin gap (ħ ω =0.25 meV). The inset shows the exciton energy versus temperature, determined from the position of the peak maximum, ħ ω max , in panel ( a ). ( c ) Comparison of the normalised resonance energies, ħω res / k B T N (or T c ), plotted versus reduced temperature, T / T N (or T c ), in CeB 6 , in several unconventional superconductors [3] , [4] , [6] , and in the low-temperature phase of CeRu 2 Al 10 (ref. 35 ). The lines are guides to the eyes. Full size image Spin gap and the Q -space structure of the INS signal Constant- Q scans at various high-symmetry points ( Fig. 3b,c ) further show a weakly energy-dependent magnetic response throughout the Brillouin zone. For T < T N , a spin gap of magnitude ~0.5 meV opens up nearly isotropically in momentum space, including the M point, where the magnetic INS signal is minimal, and the R point, where the resonant mode develops in the AFM state. The appearance of the spin gap is consistent with the depletion in the electronic density of states below T N , previously observed by point-contact spectroscopy [30] . The comparison in Fig. 4b of the temperature scans measured at the peak maximum (0.5 meV) and below it (0.25 meV) emphasises that the spectral-weight gain at the exciton energy is compensated by its depletion within the spin-gap region. Both effects show a simultaneous sharp onset at T N , closely similar to the behaviour of the resonant mode and the spin gap in an unconventional superconductor [3] . An analogous T -evolution is observed at the point ( Fig. 3c ), where a quasielastic signal of comparable intensity is found in the AFQ state. The redistribution of spectral weight at this point leads to an intensity enhancement below T N at ħω ≈ 0.9 meV, but the resulting feature is much broader than the one at the R point. Although the resonant mode is most intense at , the intensity map in Fig. 2a suggests the presence of weaker tails extending well into the Brillouin zone. This observation is substantiated by Fig. 5 , where we show momentum scans along the Λ T Λ′ ( Fig. 5a ) and Σ M Σ′ ( Fig. 5b ) directions that cut the two lobes of intensity extending from R towards the M point. The comparison of the low-temperature signals measured at 0.5 and 0.25 meV together with the energy scan at the Λ point ( Fig. 3b,c ) let us conclude that the mode exhibits at most a weak dispersion, so that even away from the R point, its intensity remains maximal near ħω max ≈ 0.5 meV. 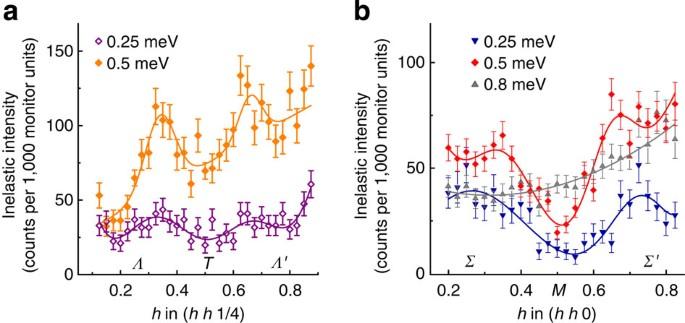Figure 5: Anisotropic shape of the resonant mode in momentum space. (a,b) Low-temperature (T=1.6 K)Q-scans along theand (hh0) directions (left and right panels, respectively) cross the two intensity lobes that connect the resonant peaks at equivalentRpoints, resulting in two incommensurate peaks. The intensity is maximised at the resonance energy (ħω=0.5 meV) and is much reduced both within the spin gap (ħω=0.25 meV) and at a higher energy (ħω=0.8 meV). The letters on the horizontal axes mark points in the Brillouin zone according to the notation inFig. 3b(inset). Figure 5: Anisotropic shape of the resonant mode in momentum space. ( a,b ) Low-temperature ( T =1.6 K) Q -scans along the and ( hh 0) directions (left and right panels, respectively) cross the two intensity lobes that connect the resonant peaks at equivalent R points, resulting in two incommensurate peaks. The intensity is maximised at the resonance energy ( ħω =0.5 meV) and is much reduced both within the spin gap ( ħω =0.25 meV) and at a higher energy ( ħω =0.8 meV). The letters on the horizontal axes mark points in the Brillouin zone according to the notation in Fig. 3b (inset). Full size image Although the quasielastic intensity in the paramagnetic state of CeB 6 is similar to the one observed in other heavy-fermion compounds [5] , [6] , the behaviour of the resonant mode we have discovered for T < T N is quite different from that of low-energy magnons in other heavy-fermion antiferromagnets, including the isostructural PrB 6 (ref. 31 ), as well as CeIn 3 (ref. 32 ) and CePd 2 Si 2 (ref. 33 ). These excitations exhibit the conventional dispersion with minimum energy and maximum intensity at the AFM-ordering wave vector. The resonant mode in CeB 6 , on the other hand, is much more intense, at most weakly dispersive, and centred at Q AFQ rather than Q AFM . The behaviour we have observed disagrees with calculations in the framework of the interacting-multipole model of CeB 6 , which predict magnon-like low-energy modes [19] , in addition to more weakly dispersive higher-energy crystal-field excitations [34] . The striking similarity of the resonant mode in CeB 6 to the low-energy spin excitations in unconventional superconductors can be qualitatively understood in the framework of a two-component model that includes strong interactions of the localised magnetic moments with the itinerant electrons [5] . The formation of the AFM state accounts for the opening of a gap in the electronic density of states near the Fermi energy, which is similar to that found in spin-density-wave systems. As a consequence, it leads to the nearly isotropic spin gap in the continuous magnetic spectrum originating from strongly hybridised crystal-field excitations of the Ce 4 f -electrons and the itinerant conduction electrons. The resonant mode can then be regarded as a collective mode below the onset of the particle-hole continuum, in close analogy to current theoretical models of the resonant modes in the superconductors. We note that this scenario is quite different from the standard interacting-multipole model of CeB 6 , according to which the magnetic response in the AFM phase is dominated by the magnetic dipole moments of the localised Ce electrons, but qualitatively consistent with other recent observations that emphasised the importance of itinerant magnetism in this system [16] , [23] , [24] , [25] , [26] . Although there is general agreement on the collective-mode nature of the resonant modes in unconventional superconductors, the mechanisms leading to their formation are still controversial [9] , [10] . It is interesting to consider our data on CeB 6 in the light of two classes of theories that describe the mode as a magnon-like excitation of localised electrons close to a magnetically ordered state, and as an excitonic bound state of itinerant electrons, respectively. A recent calculation in the framework of the former approach [9] has reproduced the temperature evolution of the magnetic response of superconducting CeCoIn 5 from an overdamped mode above T c to a resonant collective mode below T c by assuming that the super-conducting gap removes damping channels for a low-energy Ce crystal-field excitation. An analogous model in which the superconducting gap is replaced by a spin-density-wave-type gap may explain the resonant mode in CeB 6 . However, the appearance of the resonant mode at the R point rather points towards a relationship to the AFQ order, which is expected to support a soft multipolar mode at this wave vector. On the other hand, the close proximity of the resonant mode to the gap energy, which would have to be regarded as a coincidence in this approach, can be naturally explained within a scenario in which the mode is described as a weakly bound triplet exciton. The complex anisotropic shape of the collective mode in CeB 6 also suggests an influence of the fermiology of the conduction-electron system, in analogy to itinerant-electron descriptions of the resonant mode in CeCoIn 5 (ref. 10 ), and the hourglass shape of the resonant mode in the copper oxides [1] . Although such an influence is generally expected for an exciton within an itinerant-electron description, it will be interesting to explore theoretically the impact of the coherence factors on the expression for χ ″( Q , ω ) in the AFM state. This is important because the relationship between the superconducting coherence factors and the resonant mode has figured prominently in the ongoing debate about the Cooper pairing symmetry in iron pnictides [3] , [8] , [7] and heavy-fermion compounds [9] , [10] . Answers to these questions will have to await calculations that take full account of the strong coupling between the localised Ce crystal-field states and the itinerant electrons, qualitatively beyond the current interacting-multipole model of CeB 6 . The first step in this direction has been already undertaken in a recent work [35] that gives a qualitative theoretical description of the spin-exciton mode reported here in the framework of a fourfold degenerate Anderson lattice model, considering both order parameters in CeB 6 as particle-hole condensates of itinerant heavy quasiparticles. We end our discussion by noting that the resonant mode in CeB 6 apparently results from the coexistence of the AFM state with the unusual AFQ order that had remained hidden to experimental probes in zero magnetic field until the recent advent of resonant X-ray diffraction methods [20] , [21] , [22] . This unique situation explains its unusual behaviour in comparison with other heavy-fermion antiferromagnets. Presumably, as a consequence of AFQ-order fluctuations, the dynamical susceptibility at the R point of CeB 6 remains substantial even for T > T N , where the resonant mode is overdamped, and only decreases gradually upon further heating. This behaviour is reminiscent of the gradual onset of magnetic intensity in the pseudogap state of the underdoped cuprates [2] , for which various hidden order parameters have also been proposed. The mode we have observed may also be related to the higher-energy excitonic modes that have been reported in other materials with thus-far unidentified hidden order parameters, such as CeRu 2 Al 10 (ref. 36 ), and in small-gap Kondo insulators SmB 6 (ref. 37 ) and YbB 12 (ref. 38 ), whose ground states remain poorly understood. We also note that multipolar ordering phenomena have been suggested responsible for the mysterious hidden-order phase in URu 2 Si 2 , which has so far avoided direct detection by conventional solid-state probes [39] . As the 'hidden' order in CeB 6 has actually been extensively characterised, the comprehensive description of the magnetic dynamics of this compound we have initiated here will have model character for a broad class of correlated-electron materials. Sample preparation Two single-crystalline rods of Ce 11 B 6 [110] with a total mass of 8 g were prepared in a multistage process: (i) synthesis of the source powder by borothermal reduction of cerium oxide at 1,900 K in vacuum according to the routine reaction: CeO 2 +8B → CeB 6 +2BO; (ii) cold compaction of the obtained powder into rods with dimensions Ø8×60 mm and their subsequent sintering at 2,000 K; (iii) growth of the single crystals by the crucible-free inductive floating-zone melting under argon pressure in the specialised ' Crystal-111 ' equipment of the Institute for Problems of Materials Science. Taking into account high metallic conductivity of CeB 6 , its high melting point (≥ 2,823 K), and its high reactivity in the molten state, this method has proven to be the most effective for purification and growth of sufficiently large single crystals of this boride. To reduce the absorption of neutrons by the 10 B isotope, the synthesis was performed using 99.6% isotopically enriched polycrystalline 11 B powder (Ceradyne Inc., USA) with a purity of 99.96%. The purity of the initial CeO 2 (the Federal State Research and Design Institute of Rare Metal Industry, Russia) was 99.996%. The main technological parameters were: (i) crystallisation rate of 1 mm min -1 ; (ii) feed-rod rotation speed of 10 r.p.m. ; (iii) gas pressure of 0.1 MPa. The desired [110] orientation of the Ce 11 B 6 single crystals was achieved by using a correspondingly oriented seed that was prepared from a primary spontaneously grown crystal. The resulting samples had a diameter of 4–6 mm and a length of up to 50 mm. According to the spectral optical method, the concentration of impurities in the grown Ce 11 B 6 crystals did not exceed 10 −3 mass %. Data acquisition The INS data were collected using the cold triple-axis IN14 spectrometer (ILL, Grenoble, France) with a pyrolytic graphite monochromator. The sample was mounted into a standard cryostat with the (110) and (001) directions in the scattering plane. To acquire the overview maps of the reciprocal space ( Fig. 2 ), we used the Flatcone detector, equipped with Si (111) analysers that select scattered neutrons with the final momentum k f =1.40 Å −1 . In this configuration, a cold beryllium filter was installed in the path of the incident beam to eliminate the contamination from higher-order neutrons. As a consequence, the accessible energy-transfer range was restricted to 0.9 meV by the Be-filter cutoff energy. The rest of the measurements were done in the conventional triple-axis configuration with a pyrolytic graphite analyser and the Be filter installed on k f . The same fixed value of k f =1.40 Å −1 was selected. The data were corrected for the energy-dependent fraction of higher-order neutrons on the monitor. The imaginary part of the dynamical spin susceptibility, χ ″( Q , ω ), was obtained from the background-subtracted INS intensity by the fluctuation-dissipation relation , where S ( Q , ω ) is the scattering function. Reciprocal-space notation Throughout the paper, we index the reciprocal-lattice vectors on the simple-cubic unit cell (space group Pm 3 m , lattice constant a =4.1367 Å) and follow the conventional notation in labelling the high-symmetry points ( Fig. 3b , inset). The wave-vector coordinates are given in reciprocal lattice units (1 r.l.u.=2π/ a ). How to cite this article: Friemel, G. et al . Resonant magnetic exciton mode in the heavy-fermion antiferromagnet CeB 6 . Nat. Commun. 3:830 doi: 10.1038/ncomms1821 (2012).